Chromatin remodelling and autocrine TNFα are required for optimal interleukin-6 expression in activated human neutrophils Controversy currently exists about the ability of human neutrophils to produce IL-6. Here, we show that the chromatin organization of the IL-6 genomic locus in human neutrophils is constitutively kept in an inactive configuration. However, we also show that upon exposure to stimuli that trigger chromatin remodelling at the IL-6 locus, such as ligands for TLR8 or, less efficiently, TLR4, highly purified neutrophils express and secrete IL-6. In TLR8-activated neutrophils, but not monocytes, IL-6 expression is preceded by the induction of a latent enhancer located 14 kb upstream of the IL-6 transcriptional start site. In addition, IL-6 induction is potentiated by endogenous TNFα, which prolongs the synthesis of the IκBζ co-activator and sustains C/EBPβ recruitment and histone acetylation at IL-6 regulatory regions. Altogether, these data clarify controversial literature on the ability of human neutrophils to generate IL-6 and uncover chromatin-dependent layers of regulation of IL-6 in these cells. Extensive research performed in the last 20 years has contributed to the recognition of polymorphonuclear neutrophils as versatile cells linking the innate and adaptive arms of the immune response [1] . Neutrophils synthesize and release a vast repertoire of cytokines, exhibiting not only pro-inflammatory, anti-inflammatory and mitogenic actions, but also immunoregulatory activities [2] . Under many inflammatory conditions, neutrophils predominate over other cell types. Therefore, the contribution of neutrophil-derived cytokines can be of importance in determining the outcomes of infection and inflammation. Although differences in the capacity to express cytokines (for example, IL-10; ref. 3 ) between human and mouse neutrophils have been reported and debated, there is no general consensus in the literature as to whether human neutrophils produce interleukin-6 (IL-6), a cytokine displaying both pro-inflammatory and anti-inflammatory activities [4] . In some studies, IL-6 production by human neutrophils has been reported to occur constitutively, while in others no IL-6 mRNA expression has been observed in agonist-stimulated neutrophils [2] . Conflicting results have also been reported on the ability of lipopolysaccharide (LPS) to induce the accumulation of IL-6 mRNA in neutrophils, either if determined by northern blot analysis [5] , [6] , or by reverse transcription quantitative real-time PCR (RT–qPCR) [7] . Similarly, while several articles have reported the detection of remarkable amounts of IL-6 (up to 1 ng ml −1 per 24 h per 10 6 cells) in supernatants from neutrophils stimulated in vitro with LPS, granulocyte–macrophage colony-stimulating factor (GM-CSF) or other stimuli [5] , [8] , [9] , [10] , other studies indicate under similar experimental conditions that neutrophils are unable to secrete IL-6 (refs 11 , 12 ). While it should be taken into account that the experimental procedures used in all these published studies differ (for example, in terms of: neutrophil concentrations; different strains, batches, grade of purity and doses of LPS; use of human/animal serum; different time points of analysis; variable accuracy in the methods revealing IL-6 gene expression/production), the need for stringent purification procedures to control for contamination of monocytes [2] , [13] —namely, the major cellular producers of IL-6 (ref. 14 )—has rarely been met. Here we analyze, by chromatin immunoprecipitation (ChIP) assays, histone posttranslational modifications informative of the underlying chromatin state, and show that the IL-6 locus in highly purified human neutrophils has an inactive configuration. Nonetheless, Toll like receptor 8 (TLR8) agonists such as R848 and CL075 potently induce IL-6 gene expression and protein production by neutrophils, which correlate with their capacity to remodel chromatin at the IL-6 locus. Overall, these data demonstrate the existence of tight chromatin layers of regulation of IL-6 gene expression in human neutrophils. IL-6 production by human neutrophils Highly purified populations of human neutrophils (99.7±0.2%, Supplementary Fig. 1 ) [15] were incubated for up to 20 h with ultrapure LPS (upLPS; 10–10,000 ng ml −1 ; Fig. 1a,b ), or optimal stimulating doses of various agonists ( Fig. 1a–d ), including R848 (also known as resiquimod), β-glucan, curdlan, N -formyl-methionyl-leucyl-phenylalanine (fMLF), GM-CSF, tumour necrosis factor alpha (TNFα) and CpG oligodeoxynucleotides (ODN). These experiments identified R848 (an imidazoquinoline with potent antiviral activity activating immune cells via endosomal TLR7/TLR8) [16] as a potent inducer of both IL-6 mRNA ( Fig. 1a ) and protein production ( Fig. 1b ). While IL-6 transcripts were undetectable in resting neutrophils by RT–qPCR, they accumulated in R848-treated neutrophils at 3 h after stimulation and steadily increased up to 20 h ( Fig. 1a ). Extracellular IL-6 was detected after 6 h of stimulation and peaked at 20 h ( Fig. 1b ). When we used lower doses of R848 (1 μM), the profiles of IL-6 mRNA and protein were almost identical ( Fig. 1d ) but the IL-6 amounts were reduced. Such R848-mediated stimulation depended on TLR8 (refs 17 , 18 ), as revealed by the selective neutrophil expression of TLR8, but not TLR7, at both the mRNA ( Supplementary Fig. 2a ) and protein ( Supplementary Fig. 2b ) level. Moreover, a more specific TLR8 agonist, CL075 (ref. 19 ), also triggered IL-6 release, while a specific TLR7 agonist, R837 (also known as imiquimod) [20] , was inactive ( Fig. 1d ). Furthermore, R848-mediated induction of IL-6 mRNA was reproduced by using imidazoquinolines purchased from two different sources (see Methods) and abrogated by pretreatment of neutrophils with bafilomycin A1, a potent inhibitor of endosomal acidification required for efficient TLR8 signalling [21] ( Fig. 1e ). We found that neutrophil-derived IL-6 was biologically active as supernatants harvested from R848-activated neutrophils (R848-SN in Fig. 1f ) triggered, in 60 min, IL-6-dependent signal transducers and activators of transcription 3 (STAT3) tyrosine phosphorylation in human peripheral blood mononuclear cells (PBMC). Notably, a STAT3 tyrosine phosphorylation, partially dependent on endogenous IL-6, was detectable also in R848-treated PBMC starting, however, from 2 h of incubation. 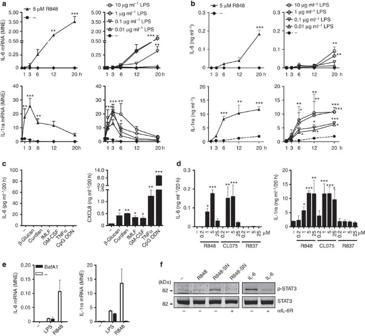Figure 1: Human neutrophils produce IL-6 in response to TLR8 or TLR4 ligands. Neutrophils (5 × 106ml−1) were cultured with either R848 (0.2–25 μM), upLPS (0.01–10 μg ml−1), particulate β-glucan (500 μg ml−1), curdlan (500 μg ml−1), fMLF (10 nM), GM-CSF (10 ng ml−1), TNFα (10 ng ml−1), CpG ODN 2006 (100 μg ml−1), CL075 (0.2–25 μM) or R837 (0.2–25 μM), for up to 20 h, to evaluate: IL-6 and IL-1ra mRNA expression by RT–qPCR (a, values represent mean±s.e.m. from 4 to 10 experiments per each time point); or IL-6 (b,n=4–22,c,n=3–15,d,n=3–22) IL-1ra (b,n=4–22,dn=3–22) and CXCL8 (c,n=3–15) protein levels, as measured by ELISA in related supernatants. (e) Neutrophils were pretreated for 30 min with 25 nM Bafilomycin A1 (BafA1) and then further incubated with 5 μM R848 or 10 μg ml−1upLPS for 5 h before measuring IL-6 and IL-1ra mRNA expression (representative experiment,n=2). (f) STAT3 tyrosine phosphorylation (as evaluated by western blot analysis) in PBMC, either untreated or cultured for 60 min with supernatants from neutrophils incubated for 20 h with 5 μM R848 or 100 ng ml−1IL-6, in the presence or absence of neutralizing IL-6R mAbs (representative experiment,n=3). Isotype control antibodies were ineffective. Gene expression data (means±s.e.m.) inaandeare depicted as mean normalized expression (MNE) units after GAPDH mRNA normalization. Asterisks indicate significant increases: *P<0.05, **P<0.01, ***P<0.001, by two-way analysis of variance (ANOVA) followed by Bonferroni’s post test (a,b) or one-way ANOVA followed by Tukey’s post test (c,d). Figure 1: Human neutrophils produce IL-6 in response to TLR8 or TLR4 ligands. Neutrophils (5 × 10 6 ml −1 ) were cultured with either R848 (0.2–25 μM), upLPS (0.01–10 μg ml −1 ), particulate β-glucan (500 μg ml −1 ), curdlan (500 μg ml −1 ), fMLF (10 nM), GM-CSF (10 ng ml −1 ), TNFα (10 ng ml −1 ), CpG ODN 2006 (100 μg ml −1 ), CL075 (0.2–25 μM) or R837 (0.2–25 μM), for up to 20 h, to evaluate: IL-6 and IL-1ra mRNA expression by RT–qPCR ( a , values represent mean±s.e.m. from 4 to 10 experiments per each time point); or IL-6 ( b , n =4–22, c , n =3–15, d , n =3–22) IL-1ra ( b , n =4–22, d n =3–22) and CXCL8 ( c , n =3–15) protein levels, as measured by ELISA in related supernatants. ( e ) Neutrophils were pretreated for 30 min with 25 nM Bafilomycin A1 (BafA1) and then further incubated with 5 μM R848 or 10 μg ml −1 upLPS for 5 h before measuring IL-6 and IL-1ra mRNA expression (representative experiment, n =2). ( f ) STAT3 tyrosine phosphorylation (as evaluated by western blot analysis) in PBMC, either untreated or cultured for 60 min with supernatants from neutrophils incubated for 20 h with 5 μM R848 or 100 ng ml −1 IL-6, in the presence or absence of neutralizing IL-6R mAbs (representative experiment, n =3). Isotype control antibodies were ineffective. Gene expression data (means±s.e.m.) in a and e are depicted as mean normalized expression (MNE) units after GAPDH mRNA normalization. Asterisks indicate significant increases: * P <0.05, ** P <0.01, *** P <0.001, by two-way analysis of variance (ANOVA) followed by Bonferroni’s post test ( a , b ) or one-way ANOVA followed by Tukey’s post test ( c , d ). Full size image In these experiments, also upLPS induced IL-6 production by neutrophils, but only after an overnight incubation and at concentrations higher than 100 ng ml −1 ( Fig. 1b ). By comparison to R848 stimulation, the amounts of LPS-induced IL-6 mRNA and protein were always lower ( Fig. 1a,b ). Similar results were observed using upLPS from different bacteria ( Escherichia coli 0111:B4, E. coli K12 or Salmonella minnesota R595) and from different commercial sources, as well as two alternative TLR4 agonists, namely lipid A (from S. minnesota R595) and shiga toxin [22] . Conversely, induction of the IL-1ra mRNA and protein by LPS and R848 were quantitatively comparable ( Fig. 1a,b ). We also observed concentrations of LPS lower than 100 ng ml −1 , although unable to induce significant IL-6, induced IL-1ra mRNA accumulation and production by neutrophils ( Fig. 1a,b ). By contrast, β-glucan, curdlan, fMLF, GM-CSF, TNFα and CpG ODN, albeit able to stimulate CXCL8 expression ( Fig. 1c ), all failed to trigger any IL-6 production in neutrophils ( Fig. 1c ). Finally, when autologous monocytes were stimulated with 5 μM R848 or 100 ng ml −1 LPS, they showed a comparatively faster kinetics of IL-6 release ( Supplementary Fig. 3a ) and mRNA expression ( Supplementary Fig. 3b ), as well as a greater capacity to respond to low doses of LPS in terms of IL-6, IL-1ra and CXCL8 production ( Supplementary Fig. 3c ). Furthermore, while kinetics of CXCL8 and CCL4 mRNA expression in neutrophils and autologous monocytes displayed different patterns, IL-10, IFNβ and CXCL10 transcripts were exclusively detected in monocytes ( Supplementary Fig. 4 ). Overall, these data demonstrate that human neutrophils efficiently produce functional IL-6 when activated with TLR8 agonists. Induction of IκBζ expression in R848-treated neutrophils To define the molecular mechanisms responsible for the activation of IL-6 expression in human neutrophils, we utilized 5 μM R848 ( Fig. 1 ). We first examined whether R848 could induce IκBζ, an inducible, atypical IκB family member and transcriptional co-activator required for the expression of a subset of inflammatory genes such as IL-6 , CSF3 and IL12b (ref. 23 ). The IL-6 gene is a secondary response gene in neutrophils, since its induction (as well as the induction of CSF3 and IL12b , but not IL-1ra ) by R848 was almost completely abolished by the protein synthesis inhibitor cycloheximide (CHX; Fig. 2a ). Consistently IκBζ protein expression was induced within 1 h of R848 treatment, peaked at 3 h and remained stable up to 20 h ( Fig. 2b ). Such a prolonged IκBζ protein expression in R848-treated neutrophils correlated not only with the sustained phosphorylation of both NF-κBp65 and mitogen-activated protein kinase (MAPK) p38 ( Fig. 2c ), but also with the kinetics of IL-6 ( Fig. 1a ), IL-12p40 and granulocyte colony-stimulating factor (G-CSF; Fig. 2d ) mRNA expression. By contrast, induction of IκBζ protein expression in R848-stimulated monocytes was transient ( Supplementary Fig. 3d ), thus correlating with the more rapid decline of IL-6 mRNA accumulation ( Supplementary Fig. 3b ). 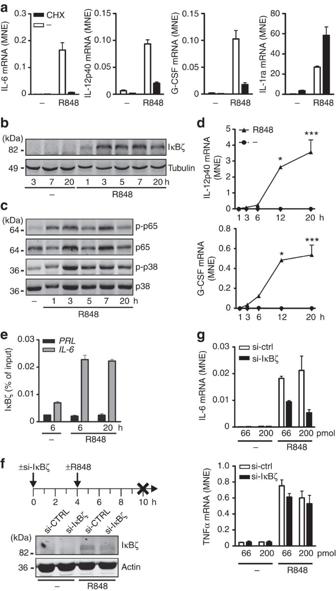Figure 2: R848 induces IκBζ expression in neutrophils. (a) IL-6, IL-12p40, G-CSF and IL-1ra mRNA expression in neutrophils preincubated with 10 μg ml−1CHX for 30 min and then cultured with 5 μM R848 for further 6 h. Induction of IκBζ expression (b) or NF-κBp65 and p38 MAPK activation (c) in neutrophils incubated with 5 μM R848 for the times indicated, as determined by western blot analysis. (d) Kinetics of IL-12p40 and G-CSF mRNA expression in neutrophils cultured with 5 μM R848 for up to 20 h (n=2–9). Asterisks indicate significant increases: *P<0.05, ***P<0.001, by two-way analysis of variance followed by Bonferroni’s post test. (e) Evaluation, by ChIP, of IκBζ recruitment to theIL-6promoter of neutrophils cultured in the presence or absence of 5 μM R848, for 6 and 20 h. Co-immunoprecipitated DNA was expressed as percent of the total input. (f,g) IκBζ silencing experiments. Neutrophils were transfected with 66 (f,g) or 200 (g) picomoles of si-IκBζ or si-ctrl and, after 4 h, incubated with or without 5 μM R848 for 6 h (scheme inf, upper panel), before analysis of IκBζ protein (f) and IL-6 and TNFα mRNA (g) expression. Representative experiments out of two (a,c,e) or three (b,f,g) independent ones with similar results, are shown. Error bars represent standard errors calculated from triplicate qPCR reactions. Figure 2: R848 induces IκBζ expression in neutrophils. ( a ) IL-6, IL-12p40, G-CSF and IL-1ra mRNA expression in neutrophils preincubated with 10 μg ml −1 CHX for 30 min and then cultured with 5 μM R848 for further 6 h. Induction of IκBζ expression ( b ) or NF-κBp65 and p38 MAPK activation ( c ) in neutrophils incubated with 5 μM R848 for the times indicated, as determined by western blot analysis. ( d ) Kinetics of IL-12p40 and G-CSF mRNA expression in neutrophils cultured with 5 μM R848 for up to 20 h ( n =2–9). Asterisks indicate significant increases: * P <0.05, *** P <0.001, by two-way analysis of variance followed by Bonferroni’s post test. ( e ) Evaluation, by ChIP, of IκBζ recruitment to the IL-6 promoter of neutrophils cultured in the presence or absence of 5 μM R848, for 6 and 20 h. Co-immunoprecipitated DNA was expressed as percent of the total input. ( f , g ) IκBζ silencing experiments. Neutrophils were transfected with 66 ( f , g ) or 200 ( g ) picomoles of si-IκBζ or si-ctrl and, after 4 h, incubated with or without 5 μM R848 for 6 h (scheme in f , upper panel), before analysis of IκBζ protein ( f ) and IL-6 and TNFα mRNA ( g ) expression. Representative experiments out of two ( a , c , e ) or three ( b , f , g ) independent ones with similar results, are shown. Error bars represent standard errors calculated from triplicate qPCR reactions. Full size image The potential role of IκBζ in positively controlling the induction of IL-6 gene in R848-treated neutrophils was supported by analysing the effects of IL-10, a cytokine known to potently modulate gene expression in neutrophils [24] . IL-10 suppressed IL-6, but not IL-1ra, mRNA accumulation ( Supplementary Fig. 5a ), as well as IL-6 production, at both 6 and 20 h of neutrophil treatment with R848, together with a partial downregulation of IκBζ mRNA ( Supplementary Fig. 5a ) and protein expression ( Supplementary Fig. 5b ). Because neutrophils, by comparison to monocytes, do not produce IL-10 when incubated with R848 (ref. 3 ), our data are in keeping with the possibility that IκBζ expression and, consequently, IL-6, G-CSF and IL-12p40 mRNA accumulation, are sustained in neutrophils because of the absence of the IL-10-mediated negative feedback pathways that control IL-6 expression in monocytes [25] . Finally, unequivocal evidence establishing that, in neutrophils, IκBζ is required for the R848-mediated induction of IL-6 mRNA expression was obtained by ChIP assays ( Fig. 2e ) and by gene silencing experiments ( Fig. 2f,g ). ChIP assays proved that IκBζ bound the IL-6 promoter in neutrophils already after 6 h of incubation ( Fig. 2e ), whereas a partial reduction of IκBζ protein expression by RNA interference ( Fig. 2f ) sufficed to strongly inhibit R848-mediated induction of IL-6, but not TNFα, mRNA accumulation ( Fig. 2g ). Transcription factor binding to the IL-6 promoter We next investigated transcriptional events at the IL-6 promoter in R848-stimulated neutrophils ( Fig. 3a ). First, IL-6 primary transcripts (PT) were induced by R848, thus confirming that IL-6 mRNA accumulation is initiated by the transcriptional induction of IL-6 . Consistently, ChIP assays demonstrated that R848 induced binding to the IL-6 promoter—schematically depicted in Fig. 3b —of the CCAAT/enhancer binding protein-β (C/EBPβ) ( Fig. 3c ), NF-κBp50 ( Fig. 3d ) and NF-κBp65 ( Fig. 3e ), three transcription factors (TFs) previously shown to transactivate IL-6 gene expression [26] . Consistent with the IL-6 transcriptional kinetics, C/EBPβ binding to the neutrophil IL-6 promoter started from 3 h after R848 treatment, and peaked at 20 h ( Fig. 3c ), while binding of NF-κBp50 and NF-κBp65 were detected, respectively, starting from 6 h ( Fig. 3d ) and only at 20 h ( Fig. 3e ). C/EBPβ, NF-κBp50 and NF-κBp65 were recruited to the CXCL8 promoter at maximal amounts within 3 h post stimulation ( Supplementary Fig. 6 ), suggesting they are rapidly activated in R848-stimulated neutrophils. Therefore, the delayed recruitment of C/EBPβ, NF-κBp50 and NF-κBp65 to the IL-6 promoter likely indicates the requirement for additional regulatory events in regulating IL-6 gene expression. 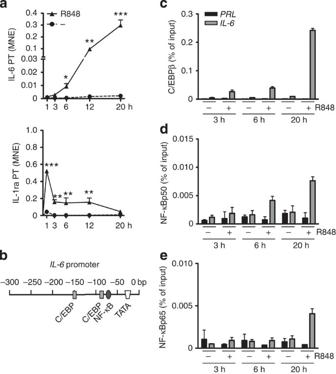Figure 3: Transcription factor recruitment to theIL-6promoter of R848-treated neutrophils. (a) IL-6 and IL-1ra primary transcript (PT) expression in neutrophils cultured with 5 μM R848 for up to 20 h (n=3–9). Asterisks indicate significant increases: *P<0.05, **P<0.01, ***P<0.001, by two-way analysis of variance followed by Bonferroni’s post test. (b) Scheme illustrating the binding sites for C/EBPβ, NF-κBp50 and NF-κBp65 at the humanIL-6promoter. Evaluation, by ChIP analysis, of C/EBPβ (c), NF-κBp50 (d) and NF-κBp65 (e) recruitment to theIL-6promoter of neutrophils cultured in the presence or absence of 5 μM R848 for up to 20 h. Co-immunoprecipitated DNA was expressed as percent of the total input. (c–e) depict a representative experiment out of three independent ones with similar results. Error bars represent standard errors calculated from triplicate qPCR reactions. Figure 3: Transcription factor recruitment to the IL-6 promoter of R848-treated neutrophils. ( a ) IL-6 and IL-1ra primary transcript (PT) expression in neutrophils cultured with 5 μM R848 for up to 20 h ( n =3–9). Asterisks indicate significant increases: * P <0.05, ** P <0.01, *** P <0.001, by two-way analysis of variance followed by Bonferroni’s post test. ( b ) Scheme illustrating the binding sites for C/EBPβ, NF-κBp50 and NF-κBp65 at the human IL-6 promoter. Evaluation, by ChIP analysis, of C/EBPβ ( c ), NF-κBp50 ( d ) and NF-κBp65 ( e ) recruitment to the IL-6 promoter of neutrophils cultured in the presence or absence of 5 μM R848 for up to 20 h. Co-immunoprecipitated DNA was expressed as percent of the total input. ( c – e ) depict a representative experiment out of three independent ones with similar results. Error bars represent standard errors calculated from triplicate qPCR reactions. Full size image Chromatin reorganization of the IL-6 locus in neutrophils As IL-6 is a secondary response gene that in macrophages requires chromatin remodelling to become accessible to the transcriptional machinery [27] , we analysed the IL-6 chromatin status by inspecting the patterns of histone posttranslational modifications in neutrophils treated or not with R848 for 6 and 20 h. As positive control, we used autologous monocytes incubated with R848 for 6 h, a time point coinciding with the peak IL-6 mRNA accumulation ( Supplementary Fig. 3b ). On the basis of the available data from genome-wide ChIP-seq of H3K4me1 in untreated PBMC and monocytes as part of the ENCODE project [28] ( Fig. 4 ), we designed nine primer sets amplifying potential regulatory regions of the IL-6 locus (indicated by numbers in the scheme of Fig. 4a , and corresponding to H3K4me1 peaks). The function of the five distal IL-6 regulatory elements was also investigated by IL-6 reporter gene assays, which revealed R848-inducible enhancer activities in each of them, three elements being characterized by high relative activity ( Fig. 4c ). These data are consistent with previous observations [29] . On the basis of these results, 66 kb of the IL-6 genomic locus (from −65.0 kb to +500 bp, relative to the transcription start site (TSS)) ( Fig. 5a ) were scanned by ChIP assays for chromatin modifications associated with active or poised genomic regulatory elements [30] , including (in addition to H3K4me1): (i) H3K4me3, which marks active promoters; (ii) H3K27Ac and (iii) H4Ac, which are enriched at active enhancers and promoters. H3K4me3 was barely detectable at the IL-6 TSS in neutrophils treated with R848 for 6 h, but was induced after 20 h ( Fig. 5b ). H3K4me3 amounts were higher in R848-treated monocytes ( Fig. 5f ), in line with the ability of these cells to robustly transcribe IL-6. Also H3K27Ac and H4Ac enrichments at the IL-6 locus of neutrophils were low at 6 h, and induced after 20 h of R848 treatment ( Fig. 5c,d ), with final amounts almost comparable to those detected in monocytes ( Fig. 5g,h ). Notably, H3K4me1 was absent at distal enhancers both before and early after stimulation (6 h), while it increased by 5- to 25-fold (depending on the region) at 20 h ( Fig. 5e ), thus indicating the emergence of latent or de novo enhancers [31] . By contrast, high levels of H3K4me1 were found already present at the same regions in unstimulated monocytes, and remained unchanged after cell activation ( Fig. 5i ). Finally, the enhancer located at 14 kb upstream of TSS (corresponding to primers #4) was found to contain high H3K4me1, H3K27Ac and H4Ac amounts only in 20 h-stimulated neutrophils (dashed boxes in Fig. 5c–e ), but not in monocytes ( Fig. 5g–i ). Conversely, enhancers located at 64 and 49 kb upstream of TSS (corresponding to primers #1 and #2) displayed higher H3K27Ac, H4Ac and H3K4me1 levels in stimulated monocytes ( Fig. 5g–i ) than in neutrophils ( Fig. 5c–e ). 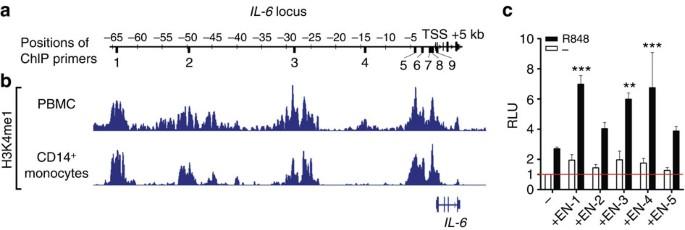Figure 4: Identification of putative regulatory sites at theIL-6locus. (a) Scheme illustrating the position of the nine primer pairs amplifying promoter and potential enhancer regions ofIL-6genomic locus that we designed for ChIP analysis (see text for explanations). Numbers above genomic locus scheme represent the distance from theIL-6transcription start site (TSS), as expressed in kilobases (kb). (b) ChIP-Seq profiles of H3K4me1 in PBMC (upper density bar) and in CD14+monocytes (lower density bar), as retrieved from ENCODE database. Since potential regulatory regions are usually associated with the peak levels of H3K4me1, we designed nine primer sets corresponding to H3K4me1 peaks (as depicted ina), with the purpose of examining the chromatin status at those regions in neutrophils and monocytes by ChIP analysis. (c) Specific enhancer activities of distalIL-6regulatory regions. pGL4-phIL6 luciferase empty construct or pGL4-phIL6 containing various enhancer regions (corresponding to 1–5, as depicted in panela) were transfected in HEK293 cells stably expressing TLR8. Cells were subsequently stimulated with 30 μM R848 for 24 h and then luciferase activities were measured and expressed as mean±s.e.m. (n=6) of relative luminescence units (RLU). Asterisks indicate significant increases: **P<0.01, ***P<0.001, by two-way analysis of variance followed by Bonferroni’s post test. Figure 4: Identification of putative regulatory sites at the IL-6 locus. ( a ) Scheme illustrating the position of the nine primer pairs amplifying promoter and potential enhancer regions of IL-6 genomic locus that we designed for ChIP analysis (see text for explanations). Numbers above genomic locus scheme represent the distance from the IL-6 transcription start site (TSS), as expressed in kilobases (kb). ( b ) ChIP-Seq profiles of H3K4me1 in PBMC (upper density bar) and in CD14 + monocytes (lower density bar), as retrieved from ENCODE database. Since potential regulatory regions are usually associated with the peak levels of H3K4me1, we designed nine primer sets corresponding to H3K4me1 peaks (as depicted in a ), with the purpose of examining the chromatin status at those regions in neutrophils and monocytes by ChIP analysis. ( c ) Specific enhancer activities of distal IL-6 regulatory regions. pGL4-phIL6 luciferase empty construct or pGL4-phIL6 containing various enhancer regions (corresponding to 1–5, as depicted in panel a ) were transfected in HEK293 cells stably expressing TLR8. Cells were subsequently stimulated with 30 μM R848 for 24 h and then luciferase activities were measured and expressed as mean±s.e.m. ( n =6) of relative luminescence units (RLU). Asterisks indicate significant increases: ** P <0.01, *** P <0.001, by two-way analysis of variance followed by Bonferroni’s post test. 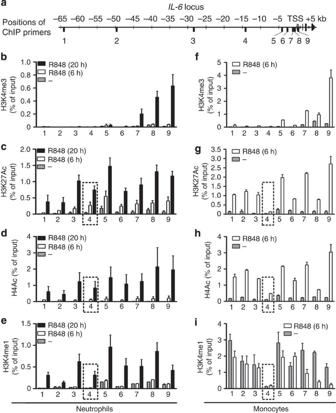Figure 5: Profiles of histone modification levels at theIL-6genomic locus of neutrophils and monocytes. (a) Scheme illustrating the positions of the nine primer pairs amplifying promoter and potential enhancer regions ofIL-6genomic locus that were designed for ChIP analysis (see text for explanations). Numbers above genomic locus scheme represent the distance from theIL-6transcription start site (TSS), as expressed in kilobases (kb). Enrichment levels of H3K4me3 (b,f), H3K27Ac (c,g), H4Ac (d,h) and H3K4me1 (e,i) by ChIP analysis in neutrophils (b–e) and in monocytes (f–i) incubated with 5 μM R848 for 6 and 20 h (neutrophils) or 6 h (monocytes). Co-immunoprecipitated DNA samples were amplified using primer pairs, as indicated inaand expressed as percent of the total input (mean±s.e.m.,n=3). Full size image Figure 5: Profiles of histone modification levels at the IL-6 genomic locus of neutrophils and monocytes. ( a ) Scheme illustrating the positions of the nine primer pairs amplifying promoter and potential enhancer regions of IL-6 genomic locus that were designed for ChIP analysis (see text for explanations). Numbers above genomic locus scheme represent the distance from the IL-6 transcription start site (TSS), as expressed in kilobases (kb). Enrichment levels of H3K4me3 ( b , f ), H3K27Ac ( c , g ), H4Ac ( d , h ) and H3K4me1 ( e , i ) by ChIP analysis in neutrophils ( b – e ) and in monocytes ( f – i ) incubated with 5 μM R848 for 6 and 20 h (neutrophils) or 6 h (monocytes). Co-immunoprecipitated DNA samples were amplified using primer pairs, as indicated in a and expressed as percent of the total input (mean±s.e.m., n =3). Full size image We next addressed the function of the increased histone acetylation at the IL-6 locus in R848-treated neutrophils. First, we detected the recruitment of two histone acetyltransferases (HATs) to the IL-6 locus of R848-treated neutrophils, namely CREB-binding protein (CBP) and, in a more delayed manner, p300 ( Supplementary Fig. 7a,b ). Second, the bromodomain-containing protein 4 (BRD4), which is recruited via interaction of its bromodomains with acetylated lysines in histones, was also inducibly recruited to the IL-6 promoter ( Supplementary Fig. 7c ). BRD4 is a member of the bromodomain and extraterminal (BET) family of chromatin readers that contribute to recruit transcription complexes to acetylated nucleosomes [32] . Given these results, we determined the effects on IL-6 induction by C646 (ref. 33 ) and HAT inhibitor II (HAT II) [34] , two selective p300/CBP inhibitors, as well as by I-BET, an inhibitor that disrupts BRD4 binding to acetylated histones [32] . We found an impairment of IL-6, but not GAPDH, mRNA induction in neutrophils incubated with R848 for 6 h ( Supplementary Fig. 7d–f ). The p300/CBP inhibitors also reduced H4Ac amounts at the IL-6 , but not GAPDH , promoter ( Supplementary Fig. 7g ). To confirm that neutrophils and monocytes use distinct enhancers at the IL-6 locus, we analysed the recruitment of PU.1 and C/EBPβ, which are known to associate with myeloid-specific regulatory regions [31] , [35] , as well as to contribute to the deposition of H3K4me1 at latent enhancers [31] , [35] . As shown in Fig. 6a,b , PU.1 and C/EBPβ were not detected in any studied regions in resting neutrophils, while they were constitutively bound to the −64, −27 and −4 kb regions (primers #1, #3 and #5) of unstimulated monocytes ( Fig. 6c,d ). However, in neutrophils treated with R848 for 6 h, PU.1 was recruited to the −27 and −4 kb regions (primers #3 and #5), at amounts comparable to monocytes ( Fig. 6a,c ). PU.1 recruitment was followed by a C/EBPβ recruitment ( Fig. 6b ), overall indicating a R848-dependent activation of these enhancer regions. While already present after 6 h of R848 treatment, and therefore before H3K4me1 deposition seen at 20 h ( Fig. 5e ), a significant recruitment of PU.1 was also exclusively found at the −14 kb region of activated neutrophils ( Fig. 6a , primers #4, dashed boxes), but not in monocytes ( Fig. 6c ), in line with their low histone modification levels at the same region ( Fig. 5g–i ). We used rVISTA software [36] on potential NF-κB binding sites in the proximity of PU.1 and used ChIP assays to show NF-κBp50 recruitment to this −14 kb enhancer site in neutrophils ( Fig. 6e ), but not in monocytes. Notably, at the IL-6 enhancer site identified at −64 kb from TSS of monocytes ( Fig. 6f , primers #1 ), ChIP assays uncovered, in addition to constitutively bound PU.1 ( Fig. 6c ) and C/EBPβ ( Fig. 6d ), the presence of high levels of interferon regulatory factor 8 (IRF8) (a TF known to mediate monocyte differentiation) [37] , thus explaining the high H3K4me1 ( Fig. 5i ). By contrast, no IRF8 signal was detected in neutrophils at the −64 kb region ( Fig. 6f ), in accordance with its absence in these cells [37] and with their lower levels of H3K4me1 ( Fig. 5e ). 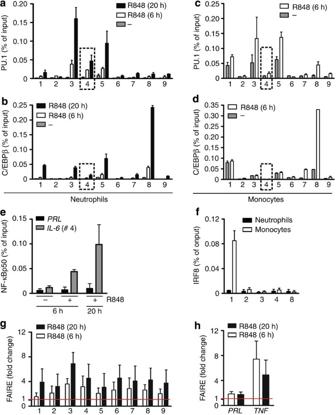Figure 6: Profiles of transcription factor binding and DNA accessibility at theIL-6genomic locus. Evaluation of PU.1 (a,c), C/EBPβ (b,d), NF-κBp50 (e) and IRF8 (f) binding to theIL-6promoter, by ChIP analysis, in neutrophils (a,b,e,f) and monocytes (c,d,f) incubated with or without 5 μM R848 for the times indicated. Co-immunoprecipitated DNA samples were amplified using primer pairs, as indicated in (Fig. 4a) and expressed as percent of the total input. Evaluation of DNA accessibility at theIL-6locus (g) orPRLandTNFpromoters (h), by FAIRE experiments, in neutrophils incubated with or without 5 μM R848 for the times indicated. Increase in DNA accessibility is displayed as fold change in activated versus resting cells. Values ina–d,g,hrepresent mean±s.e.m. (n=2–3), while values ine,fdepict a representative experiment out of three independent ones with similar results. Error bars represent standard errors calculated from triplicate qPCR reactions. Figure 6: Profiles of transcription factor binding and DNA accessibility at the IL-6 genomic locus. Evaluation of PU.1 ( a , c ), C/EBPβ ( b , d ), NF-κBp50 ( e ) and IRF8 ( f ) binding to the IL-6 promoter, by ChIP analysis, in neutrophils ( a , b , e , f ) and monocytes ( c , d , f ) incubated with or without 5 μM R848 for the times indicated. Co-immunoprecipitated DNA samples were amplified using primer pairs, as indicated in ( Fig. 4a ) and expressed as percent of the total input. Evaluation of DNA accessibility at the IL-6 locus ( g ) or PRL and TNF promoters ( h ), by FAIRE experiments, in neutrophils incubated with or without 5 μM R848 for the times indicated. Increase in DNA accessibility is displayed as fold change in activated versus resting cells. Values in a – d , g , h represent mean±s.e.m. ( n =2–3), while values in e , f depict a representative experiment out of three independent ones with similar results. Error bars represent standard errors calculated from triplicate qPCR reactions. Full size image Finally, to directly examine whether changes in chromatin accessibility occur at the IL-6 locus of neutrophils, we performed formaldehyde-assisted isolation of regulatory elements (FAIRE) [38] experiments. As shown in Fig. 6g , we found accessibility at the IL-6 locus of R848-treated neutrophils progressively increased in all the regions analysed. Instead, DNA accessibility at the TNF promoter of R848-treated neutrophils was higher at 6 h than at 20 h ( Fig. 6h ). We also found a strong enhancer RNA transcription induced in the five distal IL-6 regulatory regions of R848-treated neutrophils ( Supplementary Fig. 8 ), matching the kinetics of IL-6 primary transcript induction ( Fig. 3a ), and consistent with the activation of related enhancers [39] . Taken together, data suggest that the organization of the IL-6 locus in neutrophils and monocytes is distinct, being more closed in the former cells and more accessible in the latter ones. Nevertheless, neutrophils display the capacity to slowly reorganize the chromatin in response to R848, and, in turn, to de novo activate latent enhancers. Endogenous TNFα amplifies IL-6 expression in neutrophils We uncovered that, in neutrophils, R848 triggers a production of TNFα at much higher amounts than upLPS ( Fig. 7a ). TNFα was detected in the supernatants harvested from R848-treated neutrophils already after 3–6 h, reaching its peak after 12 h and remaining substantially stable after 20 h ( Fig. 7a ). By contrast, negligible TNFα production was measured in supernatants harvested from upLPS-treated neutrophils, being significant only at 20 h and in response to 10 μg ml −1 ( Fig. 7a ). Similarly, peak TNFα transcripts were lower in upLPS- than in R848-treated neutrophils ( Fig. 7b ). Therefore, we investigated whether endogenously produced TNFα could have a role in mediating the effect of R848 on IL-6 expression, even though exogenous TNFα fails to do so ( Fig. 1c ). Accordingly, TNFα was unable to trigger either IL-6 production ( Fig. 7c ) or IL-6 mRNA expression ( Fig. 7d ) when added to freshly isolated neutrophils at doses ranging from 0.01 to 1,000 ng ml −1 , consistent with its poor capacity to induce IκBζ mRNA and protein ( Supplementary Fig. 9 ). However, under the same conditions, TNFα upregulated IL-1ra mRNA expression and production ( Fig. 7c,d ) [2] . By using adalimumab, an anti-TNFα neutralizing antibody [40] , we found that the production of IL-6 by R848-treated neutrophils was inhibited at 20 h but not 6 h, at both the mRNA (by 61.5±4.3%, n =10, Supplementary Fig. 10 ) and protein (by 59.5±5.5%, n =18) ( Fig. 7e ) level. Likewise, adalimumab exerted a very similar inhibitory effect on R848-induced CXCL8 mRNA expression and production, but not on R848-induced IL-1ra ( Fig. 7e and Supplementary Fig. 10 ). While the results obtained with adalimumab were essentially confirmed by the use of an unrelated TNFα inhibitor, etanercept [40] , neutralizing antibodies to G-CSF, IL-6 receptor (IL-6R) or IL-1β were devoid of effects on R848-induced IL-6 production. 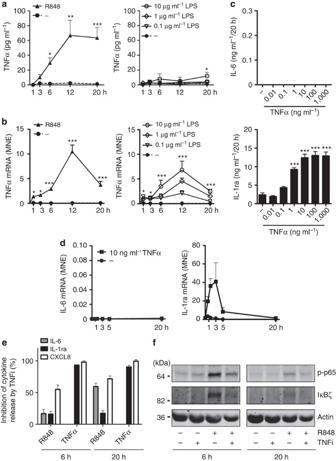Figure 7: Endogenous TNFα amplifies the induction of IL-6 in R848-stimulated neutrophils. Kinetics of TNFα release (a,n=4–22) or mRNA expression (b,n=4–10) in neutrophils cultured with R848 (5 μM) or upLPS (0.01–10 μg ml−1) for up to 20 h. (c) IL-6 and IL-1ra levels (mean±s.e.m.,n=4) in supernatants from neutrophils cultured for 20 h with or without 0.01–1,000 ng ml−1TNFα. Asterisks indicate significant increases: *P<0.05, **P<0.01, ***P<0.001, by two-way analysis of variance (ANOVA) followed by Bonferroni’s post test (a,b) and one-way ANOVA followed by Tukey’s post test (c). (d) IL-6 and IL-1ra mRNA expression, by RT–qPCR, in neutrophils cultured with 10 ng ml−1TNFα for up to 20 h. A representative experiment out of two independent ones with similar results is shown. Error bars represent standard errors calculated from triplicate qPCR reactions. (e) Neutrophils were pretreated for 30 min with 10 μg ml−1adalimumab and then incubated with 5 μM R848 or 10 ng ml−1TNFα. The levels of IL-6, IL-1ra and CXCL8 in cell-free supernatants were measured by ELISA after 6 and 20 h, and the percentage inhibition exerted by adalimumab subsequently calculated (and expressed as mean±s.e.m.,n=4–18). (f) NF-κBp65 phosphorylation and IκBζ expression (by western blot analysis) in neutrophils pretreated for 30 min with 10 μg ml−1adalimumab and then incubated with 5 μM R848 for 6 and 20 h. A representative experiment out of two independent ones with similar results is shown. Figure 7: Endogenous TNFα amplifies the induction of IL-6 in R848-stimulated neutrophils. Kinetics of TNFα release ( a , n =4–22) or mRNA expression ( b , n =4–10) in neutrophils cultured with R848 (5 μM) or upLPS (0.01–10 μg ml −1 ) for up to 20 h. ( c ) IL-6 and IL-1ra levels (mean±s.e.m., n =4) in supernatants from neutrophils cultured for 20 h with or without 0.01–1,000 ng ml −1 TNFα. Asterisks indicate significant increases: * P <0.05, ** P <0.01, *** P <0.001, by two-way analysis of variance (ANOVA) followed by Bonferroni’s post test ( a , b ) and one-way ANOVA followed by Tukey’s post test ( c ). ( d ) IL-6 and IL-1ra mRNA expression, by RT–qPCR, in neutrophils cultured with 10 ng ml −1 TNFα for up to 20 h. A representative experiment out of two independent ones with similar results is shown. Error bars represent standard errors calculated from triplicate qPCR reactions. ( e ) Neutrophils were pretreated for 30 min with 10 μg ml −1 adalimumab and then incubated with 5 μM R848 or 10 ng ml −1 TNFα. The levels of IL-6, IL-1ra and CXCL8 in cell-free supernatants were measured by ELISA after 6 and 20 h, and the percentage inhibition exerted by adalimumab subsequently calculated (and expressed as mean±s.e.m., n =4–18). ( f ) NF-κBp65 phosphorylation and IκBζ expression (by western blot analysis) in neutrophils pretreated for 30 min with 10 μg ml −1 adalimumab and then incubated with 5 μM R848 for 6 and 20 h. A representative experiment out of two independent ones with similar results is shown. Full size image We then investigated at which level anti-TNFα antibodies could interfere along the molecular cascade triggered by R848 to induce IL-6 gene expression. Adalimumab suppressed the induction of NF-κBp65 phosphorylation and IκBζ protein in R848-treated neutrophils, at both 6 and 20 h (by 62 and 32%, respectively, Fig. 7f ). Similarly, adalimumab significantly suppressed the recruitment of C/EBPβ to the IL-6 promoter in neutrophils treated with R848 at the 20 h, but not at the 6 h, time point (by 62.7±2.0%, Fig. 8a ). Furthermore, while substantially ineffective on PU.1 recruitment (neither triggered by exogenous TNFα ( Supplementary Fig. 11a )), adalimumab remarkably inhibited the increase of both H3K27Ac (between 45 and 63%, depending on the region, n =5) and H4Ac (between 47 and 63%, n =3) levels induced by R848 after 20 h at all regions of the IL-6 locus under investigation ( Fig. 8b ). Adalimumab also inhibited the increase of H3K4me1 at distal IL-6 enhancer sites starting from −14 kb region (primers #4; between 63 and 81%, n =3) but not in IL-6 promoter region ( Fig. 8b ). Altogether, these results suggest that endogenously produced TNFα sustains histone acetylation at the IL-6 promoter and surprisingly, histone methylation at the distal IL-6 enhancers, but not PU.1 recruitment, which is supposed to be the main factor responsible for H3K4me1 deposition. However, since C/EBPs were shown to collaborate with PU.1 in regulating H3K4 monomethylation at de novo formed enhancers [41] , it is likely that the effect of endogenous TNFα on H3K4me1 deposition in R848-treated neutrophils may be mediated by C/EBPβ, whose recruitment to the IL-6 promoter ( Fig. 8a ), as well as IL-6 enhancers, is strongly decreased by adalimumab. 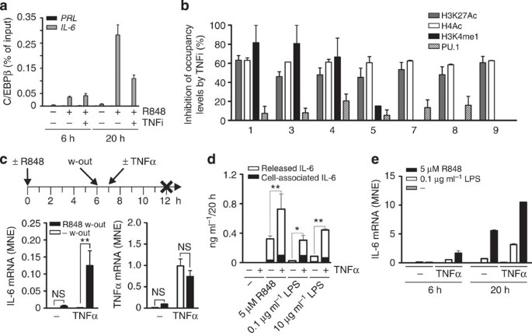Figure 8: Endogenous TNFα contributes to the reorganization of theIL-6locus in R848-stimulated neutrophils. Neutrophils were pretreated for 30 min with 5 μg ml−1adalimumab before incubation with 5 μM R848 for up to 20 h, to be processed for ChIP analysis using C/EBPβ (a) or H3K27Ac, H4Ac, H3K4me1 and PU.1 (b) Abs. For (a), precipitated DNA was amplified using primer pair #8, as indicated inFig. 4a, and expressed as percent of the total input (a representative experiment out of three independent ones with similar results is depicted and error bars represent standard errors calculated from triplicate qPCR reactions). For (b), histone modifications along the entireIL-6locus were measured using the nine primer pairs, as indicated inFig. 4a, and the percentage inhibition exerted by adalimumab calculated and expressed as mean±s.e.m. (n=3–5). (c) Neutrophils were incubated with or without 5 μM R848 for 6 h, extensively washed, and, after 1 h (to recover), cultured for an additional 5 h in the presence or the absence of 10 ng ml−1TNFα (as illustrated in the upper scheme). Extracellular IL-6 was then measured by ELISA (n=3, bottom panel inc). Asterisks indicate a significant cytokine induction by exogenous TNFα (**P<0.01, by two-way analysis of variance (ANOVA) followed by Bonferroni’s post test). NS, not significant. (d) Neutrophils were incubated for 1 h with 5 μM R848 or 0.1–10 μg ml−1upLPS before addition of 10 ng ml−1TNFα for further 20 h. IL-6 levels (shown as mean±s.e.m.,n=5) were then determined in cell-free supernatants and in corresponding cell pellets by ELISA. Asterisks indicate significant synergistic effects exerted by TNFα (*P<0.05, **P<0.01, by two-way ANOVA followed by Bonferroni’s post test). (e) IL-6 mRNA expression, by RT–qPCR, in neutrophils incubated for 1 h with 0.1 μg ml−1upLPS or 5 μM R848 followed by the addition of 10 ng ml−1TNFα for up to 20 h. A representative experiment out of three independent ones with similar results is shown. Inaandeerror bars represent standard errors calculated from triplicate qPCR reactions. Figure 8: Endogenous TNFα contributes to the reorganization of the IL-6 locus in R848-stimulated neutrophils. Neutrophils were pretreated for 30 min with 5 μg ml −1 adalimumab before incubation with 5 μM R848 for up to 20 h, to be processed for ChIP analysis using C/EBPβ ( a ) or H3K27Ac, H4Ac, H3K4me1 and PU.1 ( b ) Abs. For ( a ), precipitated DNA was amplified using primer pair #8, as indicated in Fig. 4a , and expressed as percent of the total input (a representative experiment out of three independent ones with similar results is depicted and error bars represent standard errors calculated from triplicate qPCR reactions). For ( b ), histone modifications along the entire IL-6 locus were measured using the nine primer pairs, as indicated in Fig. 4a , and the percentage inhibition exerted by adalimumab calculated and expressed as mean±s.e.m. ( n =3–5). ( c ) Neutrophils were incubated with or without 5 μM R848 for 6 h, extensively washed, and, after 1 h (to recover), cultured for an additional 5 h in the presence or the absence of 10 ng ml −1 TNFα (as illustrated in the upper scheme). Extracellular IL-6 was then measured by ELISA ( n =3, bottom panel in c ). Asterisks indicate a significant cytokine induction by exogenous TNFα (** P <0.01, by two-way analysis of variance (ANOVA) followed by Bonferroni’s post test). NS, not significant. ( d ) Neutrophils were incubated for 1 h with 5 μM R848 or 0.1–10 μg ml −1 upLPS before addition of 10 ng ml −1 TNFα for further 20 h. IL-6 levels (shown as mean±s.e.m., n =5) were then determined in cell-free supernatants and in corresponding cell pellets by ELISA. Asterisks indicate significant synergistic effects exerted by TNFα (* P <0.05, ** P <0.01, by two-way ANOVA followed by Bonferroni’s post test). ( e ) IL-6 mRNA expression, by RT–qPCR, in neutrophils incubated for 1 h with 0.1 μg ml −1 upLPS or 5 μM R848 followed by the addition of 10 ng ml −1 TNFα for up to 20 h. A representative experiment out of three independent ones with similar results is shown. In a and e error bars represent standard errors calculated from triplicate qPCR reactions. Full size image Because exogenous TNFα is unable to trigger any PU.1 ( Supplementary Fig. 11a ), or H4Ac ( Supplementary Fig. 11b ) and H3K27Ac deposition at the IL-6 locus ( Supplementary Fig. 11c ), and consequently IL-6 mRNA expression ( Fig. 7d ), it is evident that the signalling cascades activated by exogenous TNFα in neutrophils are unable to modify the chromatin status at the IL-6 locus. This was also confirmed by the FAIRE experiments, showing that exogenous TNFα fails to promote DNA accessibility at any of the IL-6 regulatory regions, in contrast to its positive effects on chromatin remodelling at the TNF promoter ( Supplementary Fig. 11d ). On the other hand, if TNFα signals in neutrophils under conditions in which the chromatin has already been modified at the IL-6 locus in response to R848 treatment, then it amplifies C/EBPβ recruitment, histone acetylation and, eventually, IL-6 gene expression. To test this, neutrophils were pretreated with or without R848 for 6 h (a time frame that, based on the results shown in Fig. 5 , is sufficient to initiate a chromatin reorganization at the IL-6 locus), then extensively washed and finally re-incubated in the presence or the absence of 10 ng ml −1 TNFα for 5 h (top scheme in Fig. 8c ). As shown in Fig. 8c , a specific induction of IL-6, but not TNFα, mRNA expression by exogenous TNFα was exclusively detected in neutrophils pretreated with R848, but not cultured in medium only. Consistently, experiments in which exogenous TNFα was added to neutrophils, with either 5 μM R848 or 0.1–10 μg ml −1 upLPS, greatly accelerated and amplified the production of IL-6 ( Fig. 8d ), as well as the induction of IL-6 transcripts ( Fig. 8e ). Importantly, such a TNFα-mediated effect was not caused by triggering IL-6 secretion from an intracellular pool produced and stored in response to R848 or LPS ( Fig. 8d ). Co-treatment of neutrophils with 10 pg ml −1 TNFα and 100 ng ml −1 upLPS was sufficient to double the amounts of extracellular IL-6 recovered after 20 h of incubation, while other stimuli such as fMLF, β-glucan, curdlan and CpG ODN confirmed their incapacity to upregulate IL-6 gene expression even if co-delivered with R848 or LPS. Altogether, data provide evidence that, in neutrophils incubated with R848, specific chromatin changes occur at the IL-6 locus, which ultimately promote the responsiveness to endogenous TNFα in terms of IL-6 expression induction. IL-6 production by murine neutrophils in vitro and in vivo Finally, we investigated whether murine neutrophils produce IL-6 in response to R848. As shown in Fig. 9a,b , inflammatory peritoneal neutrophils, isolated by cell sorting to 99.5% purity ( Supplementary Fig. 12 ), were found to express IL-6 mRNA and to produce IL-6 when cultured for 14 h in vitro with 25 μΜ R848 or 10 μg ml −1 LPS. By contrast, no IL-6 was measured in supernatants from bone marrow-derived neutrophils cultured under the same conditions, confirming previous findings [42] . In line with these results, only inflammatory peritoneal, but not bone marrow, neutrophils were found to express TLR7 and TLR8 mRNA ( Fig. 9c ). Similar to human neutrophils ( Fig. 8d ), R848-triggered de novo IL-6 synthesis in murine neutrophils was followed by its complete extracellular release, as previously shown in response to bacteria [43] . 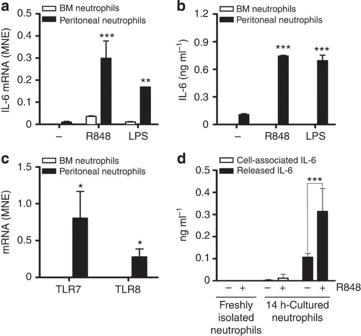Figure 9: Peritoneal inflammatory neutrophils produce IL-6 in response to R848. Murine neutrophils, isolated by cell sorting (Supplementary Fig. 12) from bone marrow or inflamed peritoneum, were either incubated with or without 25 μM R848 or 10 μg ml−1LPS for 14 hin vitro(a,b), or directly lysed (c) for evaluation of IL-6 (a), TLR7 and TLR8 (c) mRNA expression, or IL-6 release (b). (d) Mice were intraperitoneally injected first with BIOgel polyacrylamide beads, and, after 4 h, with 3 μg g−1body weight of R848 or its diluent. After 12 h, neutrophils were purified by cell sorting and either immediately processed, or cultured for 14 hin vitro. Quantification of cell-associated or released IL-6 protein was then performed by ELISA. Asterisks indicate significant increases: *P<0.05, **P<0.01, ***P<0.001, by two-way analysis of variance followed by Bonferroni’s post test. Figure 9: Peritoneal inflammatory neutrophils produce IL-6 in response to R848. Murine neutrophils, isolated by cell sorting ( Supplementary Fig. 12 ) from bone marrow or inflamed peritoneum, were either incubated with or without 25 μM R848 or 10 μg ml −1 LPS for 14 h in vitro ( a , b ), or directly lysed ( c ) for evaluation of IL-6 ( a ), TLR7 and TLR8 ( c ) mRNA expression, or IL-6 release ( b ). ( d ) Mice were intraperitoneally injected first with BIOgel polyacrylamide beads, and, after 4 h, with 3 μg g −1 body weight of R848 or its diluent. After 12 h, neutrophils were purified by cell sorting and either immediately processed, or cultured for 14 h in vitro . Quantification of cell-associated or released IL-6 protein was then performed by ELISA. Asterisks indicate significant increases: * P <0.05, ** P <0.01, *** P <0.001, by two-way analysis of variance followed by Bonferroni’s post test. Full size image On the basis of these results, we injected mice intraperitoneally first with BIOgel polyacrylamide beads for 4 h and then with 3 μg g −1 body weight of R848 or its diluent. After an additional 12 h, neutrophils were purified and either processed for total RNA extraction/cell lysis, or cultured in vitro for 14 h. As shown in Fig. 9d , the yields of extracellular IL-6 were much higher in supernatants from BIOgel/R848-elicited peritoneal neutrophils than in supernatants from control cells. Interestingly, neither intracellular IL-6 ( Fig. 9d ), nor IL-6 mRNA, were detectable in either untreated or R848-treated BIOgel-elicited peritoneal neutrophils, in line with previous studies demonstrating that murine neutrophils are induced to release IL-6 in vivo without newly accumulating IL-6 mRNA [44] . Altogether, these data demonstrate that R848 can potently induce IL-6 production by murine neutrophils not only in vitro , but also in vivo . IL-6 is a multifunctional cytokine produced by a variety of cells that has both pro- and anti-inflammatory activities [4] . More recently, IL-6 has been identified as a decisive cytokine for the differentiation of CD4 + T cells into Th17 cells, which are currently considered as a major T-cell population endowed with pro-inflammatory activities [45] . It follows that blockade of IL-6/IL-6 signalling has a profound effect on innate and acquired immune responses. Thereby, a complete understanding of how IL-6 is regulated in different cell types at the molecular level has implications for understanding not only inflammatory disease pathogenesis, but also for immunotherapeutic strategies. In such regard, the literature on human neutrophils as potential IL-6-producing cells is, to date, confusing and contradictory [2] , [5] , [8] , [9] , [10] , [11] , [12] . Using highly purified (>99.7%) cell populations, we show that human neutrophils produce biologically active IL-6 if appropriately stimulated. Specifically, we identified R848 and CL075, two selective agonists of TLR8, an endosomal receptor for single strand RNA of viral or bacterial origin [16] , as potent inducers of IL-6 mRNA expression and production in human neutrophils. Accordingly, supernatants from neutrophils activated for 20 h with R848 triggered a noticeable STAT3 tyrosine phosphorylation in human PBMC, such an effect being completely inhibited by neutralizing antibodies to IL-6R. By contrast, well-known neutrophil agonists, such as β-glucan, curdlan, fMLF, GM-CSF, TNFα and CpG ODN, even when used at maximal stimulatory concentrations, were found to be unable to induce IL-6 mRNA expression or production by neutrophils. Corroborating the results on human cells, we ascertained that R848 induces IL-6 production also in murine neutrophils, not only in vitro , but also in vivo . Characterization of the molecular bases underlying R848-induced IL-6 production in human neutrophils uncovered that R848 induces a sequence of time-dependent events occurring at the chromatin level. ChIP analysis of posttranslational modifications of histones associated with genes that are active or poised for transcriptional activation, including H3K4me3, H4Ac, H3K27Ac and H3K4me1 marks [30] indicated the chromatin status of the IL-6 genomic locus in freshly isolated neutrophils to be inactive, whereas in autologous monocytes the status appeared already ‘poised’ for transcription and more prone for rapid chromatin remodelling. Curiously, similar chromatin signatures were previously identified in both neutrophils and monocytes in the case of the IL-10 locus [46] . However, while in neutrophils the IL-10 locus remains inaccessible and inactive regardless of their stimulation (including with R848) [46] , the IL-6 locus undergoes a slow, but extensive, chromatin reorganization upon TLR8 engagement (as schematically illustrated in Fig. 10 ). Moreover, while neutrophils rearranged an IL-6 enhancer site located in the 14 kb upstream of IL-6 TSS, monocytes preferentially reorganized a different IL-6 enhancer at −64 kb from the IL-6 TSS (see scheme in Fig. 10 ). 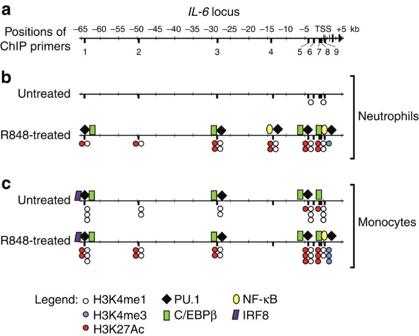Figure 10: Chromatin reorganization at theIL-6locus of neutrophils and monocytes treated with R848. (a) Same scheme displayed inFig. 4a. (b,c) Scheme illustrating the occupancy of PU.1, NF-κB, C/EBPβ and IRF8, as well as H3K4me1, H3K4me3 and H3K27Ac at the various regulatory regions of theIL-6locus of neutrophils (b) and monocytes (c), before (upper bars, indicated as ‘untreated’) and after (lower bars, indicated as ‘R848-treated’) incubation with R848 for 20 h (b) or 6 h (c). The degree of each histone modification enrichment in each region is represented by the number of distinctively coloured circles. The scheme illustrates that theIL-6locus of untreated neutrophils is inactive based on the absence of histone modifications and TF binding (b, upper bar). Upon neutrophil treatment with R848, recruitment of PU.1, C/EBPβ, NF-κB and deposition of significant levels of histone marks (H3K27Ac, H3K4me1, H3K4me3) occur at variousIL-6locus positions (b, lower bar), suggesting an induction of latent regulatory sites leading toIL-6gene transcription. By contrast, constitutively bound PU.1, C/EBPβ and IRF8, associated with significant levels of H3K4me1 at readily responsiveIL-6enhancers in resting monocytes (c, upper bar), stand for an already-poised state of the monocyteIL-6locus. Upon monocyte treatment with R848, only acetylation atIL-6enhancers, as well as TF recruitment and H3K4me3 deposition atIL-6promoter are triggered (c, lower bar), thereby leading to a rapid transcriptional activation of theIL-6locus. Figure 10: Chromatin reorganization at the IL-6 locus of neutrophils and monocytes treated with R848. ( a ) Same scheme displayed in Fig. 4a . ( b , c ) Scheme illustrating the occupancy of PU.1, NF-κB, C/EBPβ and IRF8, as well as H3K4me1, H3K4me3 and H3K27Ac at the various regulatory regions of the IL-6 locus of neutrophils ( b ) and monocytes ( c ), before (upper bars, indicated as ‘untreated’) and after (lower bars, indicated as ‘R848-treated’) incubation with R848 for 20 h ( b ) or 6 h ( c ). The degree of each histone modification enrichment in each region is represented by the number of distinctively coloured circles. The scheme illustrates that the IL-6 locus of untreated neutrophils is inactive based on the absence of histone modifications and TF binding ( b , upper bar). Upon neutrophil treatment with R848, recruitment of PU.1, C/EBPβ, NF-κB and deposition of significant levels of histone marks (H3K27Ac, H3K4me1, H3K4me3) occur at various IL-6 locus positions ( b , lower bar), suggesting an induction of latent regulatory sites leading to IL-6 gene transcription. By contrast, constitutively bound PU.1, C/EBPβ and IRF8, associated with significant levels of H3K4me1 at readily responsive IL-6 enhancers in resting monocytes ( c , upper bar), stand for an already-poised state of the monocyte IL-6 locus. Upon monocyte treatment with R848, only acetylation at IL-6 enhancers, as well as TF recruitment and H3K4me3 deposition at IL-6 promoter are triggered ( c , lower bar), thereby leading to a rapid transcriptional activation of the IL-6 locus. Full size image The identification of endogenously produced TNFα as amplifier of IL-6 production in R848-stimulated neutrophils further illustrates how sophisticated and cell-specific is the control of the IL-6 gene expression in myeloid cells. Accordingly, unlike exogenous TNFα alone—which was unable to increase chromatin accessibility at the IL-6 locus and consequently to induce IL-6 gene expression—endogenously produced TNFα increased histone acetylation as well as deposition of H3K4me1 at distal enhancer sites of the IL-6 locus. Furthermore, at delayed times of incubation, endogenously produced TNFα also sustained IκBζ protein expression and C/EBPβ recruitment, because it operates in cells in which the IL-6 locus has already undergone a reorganization following R848 stimulation. Altogether, these data indicate that IL-6 expression in human neutrophils is prominently and dynamically regulated at the chromatin level, with the contribution of effects mediated by endogenously produced TNFα. More broadly, our results also indicate that the quality of responsiveness to TNFα by neutrophils may change depending on how signals present in the microenvironment specifically modify their chromatin status. Such a phenomenon might be important, for instance, in the context of anti-TNFα treatment. We also showed that, although less efficiently than TLR8 agonists, TLR4 ligands, including upLPS from various bacteria, lipid A and shiga toxin [22] , do trigger IL-6 mRNA expression and production by highly purified populations of neutrophils, but only if used at concentrations higher than 100 ng ml −1 and after an overnight incubation. Our data thus clarify the many contrasting results reported by the literature related to the issue of whether or not LPS-stimulated human neutrophils express/produce IL-6 (refs 8 , 9 , 10 , 11 , 12 ). As highlighted by numerous experimental and molecular evidence provided herein, including an accurate comparison with autologous monocytes, it is our speculation that all studies reporting that TLR4-stimulated neutrophils express IL-6 mRNA at times shorter than 5-6 h, and/or produce IL-6 before 6 h of incubation at levels higher than 200 pg ml −1 per 5 × 10 6 cells, are likely influenced by monocyte contamination [11] . Our observations on the molecular bases whereby human neutrophils treated with TLR8 agonists produce IL-6 expand our knowledge on the range of effects R848, CL075 and other TLR8-related ligands exert on neutrophils. These comprise cell shape changes, CD62L shedding, priming for enhanced respiratory burst [17] , [47] , [48] , [49] , chemotaxis, phagocytosis [17] , [50] and neutrophil extracellular trap formation induction [51] , lipid mediator production [18] , prolonged survival [49] , [52] and cytokine production (using, however, less pure neutrophil populations than in this study), including TNFα [53] and IL-6 (refs 48 , 53 , 54 ). Similarly, two studies [55] , [56] have reported that human neutrophils cultured in the presence of infectious respiratory syncytial virus produce IL-6 at 1 ng ml −1 per 5 × 10 6 cells per 3 h (>98% neutrophil purity [55] ), or at 100 pg ml −1 per 5 × 10 5 cells per 12 h (>97% purity [56] ). Even though these data require corroboration using highly purified neutrophils, it is likely that, being a single-stranded RNA virus, respiratory syncytial virus activates neutrophil TLR8 to ultimately induce IL-6 expression. In this context, recent findings are not only reevaluating the role of neutrophils in fighting viral infections [57] but also have uncovered that neutrophils express a broad repertoire of functional cytoplasmic pattern-recognition receptors involved in the recognition of nucleic acids of viral and bacterial origin [58] , [59] . Considering that agonists of TLR8, including R848, are currently being considered as promising antiviral and anticancer drugs [60] , our data imply that neutrophils may participate in the therapeutic/side effects of these drugs via IL-6/TNFα production. Cell purification and culture Granulocytes were isolated and manipulated under endotoxin-free conditions from buffy coats of healthy donors. Briefly, after Ficoll-Paque gradient centrifugation of buffy coats, followed by dextran sedimentation of granulocytes and hypotonic lysis of erythrocytes, neutrophils were isolated to reach 99.7±0.2% purity ( Supplementary Fig. 1a ) by positively removing any eventual contaminating cells using the EasySep neutrophil enrichment kit (StemCell Technologies, Vancouver, Canada) [15] . Human monocytes were isolated from PBMCs, after Ficoll-Paque gradient centrifugation of buffy coats, by anti-CD14 microbeads (Miltenyi Biotec, Bergisch Gladbach, Germany) to reach >98% purity ( Supplementary Fig. 1b ). Neutrophils and monocytes were then suspended at 5 × 10 6 ml −1 and 2.5 × 10 6 ml −1 , respectively, in RPMI 1640 medium supplemented with 10% low-endotoxin fetal bovine serum (<0.5 EU ml −1 ; from BioWhittaker-Lonza, Basel, Switzerland), treated or not with 0.001–100 μg ml −1 upLPS from E. coli 0111:B4 strain (from either Alexis, Enzo Life Sciences, Farmingdale, NY, USA, or InvivoGen, San Diego, CA, USA), E. coli K12 strain, S. minnesota R595 strain, 0.1–10 μg ml −1 Monophosphoryl Lipid A from S. minnesota R595 (all from InvivoGen), shiga toxin (kindly provided by Professor Maurizio Brigotti, University of Bologna, Italy), 0.2–50 μM R848, CL075 or R837 (InvivoGen and Enzo Life Sciences), 100 μg ml −1 CpG ODN 2006 (InvivoGen), 0.01–1,000 ng ml −1 TNFα, 100 ng ml −1 IL-6 (Peprotech, Rocky Hill, NJ, USA, and/or R&D Systems, Minneapolis, MN, USA), 10 ng ml −1 GM-CSF (Miltenyi Biotec), 10 nM fMLF (Sigma, Saint Louis, MO, USA), 500 μg ml −1 particulate β-glucan (InvivoGen), 500 μg ml −1 curdlan (Sigma) and then plated either in 6- or 24-well tissue culture plates or in polystyrene flasks from Greiner Bio-One (Kremsmünster, Austria) for culture at 37 °C, 5% CO 2 atmosphere for the indicated times. In selected experiments, neutrophils or PBMC were preincubated for 30 min with 10 μg ml −1 cycloheximide (CHX) (Sigma), 25 nM Bafilomycin A1 (Merck-Millipore, Darmstadt, Germany), 100 U ml −1 IL-10 (kindly provided by Dr Rene de Waal Malefyt, Merck Research Laboratories, Palo Alto, CA, USA), 10 μg ml −1 anti-human IL-6R mAb (R&D Systems), 10 μg ml −1 adalimumab (Humira, Abbott Biotechnology Limited, Barceloneta, Puerto Rico) or etanercept (Enbrel, Amgen, Thousand Oaks, CA, USA) before cell stimulation. In other experiments, neutrophils were incubated for 2 h with or without 5 μΜ R848 before the addition of 30 or 100 μΜ C646 (Sigma), 20 or 40 μΜ HAT II (Merck-Millipore), or 0.1, 0.5 or 1 μΜ I-BET (Merck-Millipore) for additional 4 h. After the desired incubation period, neutrophils and monocytes were either processed for ChIP experiments or, for other assays, collected and spun at 300 g for 5 min. In the latter case, the resulting supernatants were immediately frozen in liquid nitrogen and stored at −80°C, while the corresponding pellets were either extracted for total RNA or lysed for protein analysis. IκBζ silencing Transfection of siRNA was performed by electroporation, using the Human Monocyte Nucleofector kit and the Amaxa Nucleofector II device (Lonza). Briefly, 15 × 10 6 neutrophils were resuspended in 100 μl nucleofector solution (included in the Nucleofector kit) containing either 66 or 200 pmol of ON-TARGETplus Human NFKBIZ (64332) siRNA pool or of ON-TARGETplus non-targeting siRNA pool (GE Healthcare Dharmacon, Lafayette, CO, USA) and then transferred to a nucleoporation cuvette. Electroporation was performed using the Y001 program of the Nucleofector II device. Transfected cells were plated in ‘recovery’ medium (IMDM supplemented with 2 mM glutamine and 10% FCS) for 4 h and, after medium replacement, were then incubated with or without 5 μM R848 for further 6 h. Transfected siRNA did not elicit any nonspecific response in neutrophils, as assessed by the lack of interferon-stimulated genes induction [61] . Flow cytometry For phenotypic studies [15] , 10 5 freshly isolated neutrophils and monocytes were centrifuged and suspended in 50 μl PBS containing 10% complement-inactivated human serum (for Fc receptor blocking). Neutrophils were then stained for 15 min at room temperature with 1:25 Vioblue anti-human CD14 (clone TÜK), 1:25 PE-Vio770 anti-human CD3 (clone BW 264156), 1:25 PE-Vio770 anti-human CD19 (clone LT19), 1:25 PE/Cy7 anti-human CD56 (clone HCD56, BioLegend, San Diego, California, USA), 1:50 brilliant Violet 510 anti-human CD45 (clone H130), 1:25 FITC anti-human CD66b (clone G10F5), 1:50 PerCP-Cy5.5 anti-human CD16 (clone 3G8), while monocytes were stained with 1:25 Vioblue anti-human CD11c (clone MJ4-27G12, Miltenyi Biotec) and 1:25 APC anti-human CD14 (clone TÜK), antibodies. For intracellular staining, 30 μl of buffy coats were initially stained at room temperature for CD14 (clone TÜK, 1:25 dilution) and CD16 (clone 3G8, 1:25 dilution). Then, after hypotonic lysis of erythrocytes, cells were fixed with 4% paraformaldehyde (Sigma), treated with 100 μl permeabilizing solution containing 0.5% saponin (Sigma) and 5% human serum (Sigma), and finally incubated with 1:30 PE anti-human TLR7 rAb (IMG-665D), 1:100 PE anti-human TLR8 mouse mAb (IMG-321D), 1:30 control rabbit IgG (20304D), all from Imgenex (San Diego, CA, USA) or 1:10 control mouse IgG 1 (BD Biosciences, San Jose, CA, USA) for 1 h on ice. Sample fluorescence was measured by a seven-colour MACSQuant Analyzer (Miltenyi Biotec). Data analysis was performed using FlowJo software Version 8.8.6 (Tree Star, Ashland, OR, USA). Enzyme-linked immunosorbent assay Cytokine concentrations in cell-free supernatants and cell-lysates were measured by enzyme-linked immunosorbent assay (ELISA) kits, specific for human IL-6 (either from Immunotools GmbH, Friesoythe, Germany, or eBioscience, San Diego, CA, USA), TNFα (eBioscience), IL-1ra (R&D Systems, Minneapolis, MN, USA), CXCL8 (Immunotools) or murine IL-6 (R&D Systems). Detection limits of these ELISAs were: 3 (Immunotools) or 8 pg ml −1 (eBioscience) pg ml −1 for IL-6, 4 pg ml −1 for TNFα, 40 pg ml −1 for IL-1ra, 16 pg ml −1 for CXCL8 and 16 pg ml −1 for murine IL-6. Reverse transcription quantitative real-time PCR One microgram total RNA, usually extracted by the RNeasy mini kit (Qiagen, Venlo, Limburg, Netherlands) from 5 × 10 6 neutrophils or 10 6 monocytes, respectively, was reverse transcribed for RT–qPCR and PT RT–qPCR analyses [7] using gene-specific primer pairs (Life Technologies, Carlsbad, CA, USA) available in the public database RTPrimerDB ( http://medgen.ugent.be/rtprimerdb ) under the following entry codes: GAPDH (3539), IL-1ra (3544), PT-IL-1ra (3650), TNFα (3551), CXCL8 (3553), IL-6 (3545), IL-10 (8230), IFNβ (3542), PT-IL-6 (8687), IκBζ (8688), IL-12p40 (3543), G-CSF (8615), TLR4 (8686), TLR7 (8684), TLR8 (8685), CXCL10 (3537) and CCL4 (3535), for human; GAPDH (8299), IL-6 (8768), TLR7 (8766) and TLR8 (8767) for murine. Data were calculated by Q-Gene software ( http://www.gene-quanti fication.de/download.html) and expressed as mean normalized expression units after GAPDH normalization. Immunoblots Whole-cell proteins were obtained from protein-rich flow-through solutions after the first centrifugation step using the RNeasy mini kit (Qiagen) for total RNA extraction procedure (see above). After an overnight incubation at −20°C, protein precipitates from the flow-through solutions were washed with pre-chilled 100% ethanol [62] , solubilized in Laemmli sample buffer and then subjected to immunoblots by standard procedures using the following antibodies: 1:500 anti-IκBζ rabbit pAbs (♯9244S), 1:1,000 anti-phospho-NF-κBp65 (Ser536) (♯3031), 1:1,000 anti-phospho-STAT3(Ser536) (♯9131), 1:1,000 anti-phospho-p38MAPK (♯9211), 1:1,000 anti-native p38 MAPK (♯9212) and 1:1,000 mouse mAb anti-native STAT3 (♯9139), all from Cell Signaling (Beverly, MA, USA), 1:500 rabbit pAb anti-NF-κBp65 (sc-372, Santa Cruz Biotechnology, Dallas, TX, USA), and 1:2,000 rabbit pAb anti-actin (A5060) and 1:2,000 mAb anti-β-tubulin (T5293) from Sigma. Blotted proteins were detected and quantified using the Odyssey infrared imaging system (LI-COR Biosciences, Lincoln, NE, USA) [25] . Immunoblot images in Figs 1 , 2 and 7 and Supplementary Figs 3, 5 and 9 have been cropped for presentation. Full size images are presented in Supplementary Fig. 13 . Chromatin immunoprecipitation assays After stimulation, cells were fixed using 1% formaldehyde for 6 min followed by 0.125 M glycine to stop the crosslinking reaction. After 6 min, ice-cold PBS was added to the flasks and cells were scraped on ice, washed three times with PBS and then lysed for 10 min in L1 buffer (50 mM Tris, pH 8.0, 2 mM EDTA, 0.1% Nonidet P-40 and 10% glycerol) supplemented with proteases (5 μg ml −1 leupeptin, 5 μg ml −1 pepstatin and 1 mM PMSF) and phosphatase inhibitors (1 mM Na 3 VO 4 , 20 μM PAO and 50 mM NaF). Nuclei were pelleted at 1,000 g in a cold microfuge and resuspended in L2 buffer (50 mM Tris, pH 8.0, 5 mM EDTA and 1% SDS plus inhibitors). Chromatin was then sheared by sonication (six rounds of 15 s pulses each, at 50% of the maximum potency of Bandelin Sonopuls HD 2070 ultrasonic homogenizer (Bandelin, Berlin, Germany)), centrifuged to pellet debris and finally 10 × diluted in dilution buffer (50 mM Tris, pH 8.0, 0.5% Nonidet P-40, 0.2 M NaCl and 5 mM EDTA). Nuclear extracts from 2.5 × 10 6 (for ChIP targeting histone modifications) or 10 7 (for ChIP targeting TFs) neutrophils and monocytes were immunoprecipitated with 1 μl anti-H3K4me3 rabbit mAbs (17-614), 1 μl anti-H4Ac pAbs (06-866) (Merck-Millipore), 1 μl anti-H3K4me1 (ab8895) and 1 μl anti-H3K27Ac (ab4729) (Abcam, Cambridge, UK), 4 μl anti-PU.1 (sc-352), 2.5 μl anti C/EBPβ (sc-150), 5 μl anti-NF-κBp50 (sc-7178), 5 μl anti-NF-κBp65 (sc-372) (Santa Cruz Biotechnology) or 5 μl anti-IRF8 (generated in-house towards amino acids 146–162 of murine protein). The co-immunoprecipitated material was then subjected to qPCR analysis using specific primers (purchased from Life Technologies), either spanning the human IL-6 locus or the CXCL8 promoter (as listed in Supplementary Table 1 ). Data from qPCR were expressed as percentage over input DNA and is displayed as means±s.e.m. To establish the background levels of ChIP experiments, the various histone modifications were quantified also at the promoter of prolactin ( PRL ) since it is completely silent in myeloid cells [63] . For IκBζ, p300, CBP and BRD4, we performed two-step crosslinking ChIP assays [64] , which, differently from the ChIP procedure described above, includes a preliminary protein–protein crosslinking step using 2 mM Di(N-succinimidyl) glutarate (Sigma) for 45 min. Nuclear extracts were then immunoprecipitated using 5 μl anti-IκBζ (♯9244S) (Cell Signaling), 5 μl anti-p300 (sc-585), 5 μl CBP (sc-369) (Santa Cruz Biotechnology) or 0.5 μl anti-BRD4 (HPA015055) rabbit pAbs (Sigma). Formaldehyde-assisted isolation of regulatory elements FAIRE experiments were performed as already described [38] , with some modifications. Briefly, after stimulation, 10 7 cells were fixed by 1% formaldehyde for 10 min, followed by 0.125 M Tris (pH 7.6) to stop the crosslinking reaction. After 6 min, ice-cold PBS was added to the flasks and cells were scraped on ice, washed three times with PBS and then lysed for 10 min in 1 ml LB1 buffer (50 mM HEPES-KOH, pH 7.5, 140 mM NaCl, 1 mM EDTA, 10% glycerol, 0.5% NP-40, 0.25% Triton X-100) supplemented with proteases and phosphatase inhibitors). Nuclei were then pelleted at 1,000 g in a cold microfuge, resuspended in 1 ml LB2 buffer (10 mM Tris–HCl, pH 8.0, 200 mM NaCl, 1 mM EDTA, 0.5 mM EGTA plus inhibitors) and gently rocked at room temperature for 10 min. Nuclei were pelleted at 1,000 g in a cold microfuge and lysed in 650 μl LB3 buffer (10 mM Tris–HCl, pH 8.0, 100 mM NaCl, 1 mM EDTA, 0.5 mM EGTA, 0.1% Na-Deoxycholate, 0.5% N-lauroylsarcosine plus inhibitors). Chromatin was then sheared by sonication (eight rounds of 15 s pulses each, at 50% of the maximum potency of Bandelin Sonopuls HD 2070 ultrasonic homogenizer) and 65 μl 10% Triton X-100 was then added to the sonicated lysates. After centrifugation to pellet nuclear debris, 10% of the sample volume was removed and de-crosslinked to measure input DNA. Subsequently, nucleosome-free DNA was phenol–chloroform extracted from both crosslinked nuclear lysates and de-crosslinked input DNA. qPCR analysis was then performed using specific primers (either spanning the human IL-6 locus or the TNF promoter, Supplementary Table 1 ). FAIRE experiments on PRL promoter were used as background of the DNA accessibility signal. qPCR data are expressed as percentage over de-crosslinked input DNA and are displayed as fold increase of activated versus resting cells. IL-6 construct preparation and luciferase reporter assays Plasmids containing the genomic regions of the IL-6 locus, numbered as 1, 2, 3 and 5 according to the scheme in Fig. 4a (or indicated as EN-1, EN-2, EN-3 and EN-5 in Fig. 4c ), were kindly provided by Dr Lionel Ivashkiv [29] . The genomic region numbered as 4 in Fig. 4a was instead generated by PCR ( Supplementary Table 2 ). The five genomic regions were then sub-cloned—by KpnI and SacI restriction sites—into the pGL4-phIL6 luciferase reporter vector, containing 1,300 bp of the IL-6 human promoter (RDB#7313, from RIKEN Bio-Resource Center, Tsukuba, Japan). 40 × 10 3 HEK293XL/TLR8 cells (InvivoGen) have been then transfected with a mixture of 0.2 μl Lipofectamine 2000 reagent (Life Technologies), 10 ng phRL-null and 100 ng of each plasmid DNA construct. After an overnight incubation, cells were washed and treated with 30 μM R848 for 24 h before assaying both firefly and renilla luciferase activities by the Dual-Glo Luciferase Assay System (Promega, Madison, WI, USA). The enzymatic activities of both luciferases were quantified using a Victor [3] multilabel plate counter (Perkin Elmer, Waltham, MA, USA). Firefly luciferase activity was normalized by Renilla luciferase activity and expressed as fold change relative to the value of the pGL4-phIL6 empty control. IL-6 production by murine neutrophils C57BL/6J mice were intraperitoneally injected with 2% (w/v) BIOgel polyacrylamide beads (Bio-Rad, Hercules, CA, USA). After 16 h, cells were isolated from peritoneal lavages [65] , stained with APC Cy7-conjugated anti-mouse CD11b (M1/70), APC-conjugated anti-mouse Ly6G (1A8) and Brilliant Violet 421-conjugated anti-mouse CD45 (30-F11) antibodies (BioLegend), and then suspended in PBS containing 2 mM EDTA and 2% fetal bovine serum before cell sorting using a high-speed sorter (FACSAriaIITM; Becton Dickinson, Franklin Lakes, NJ, USA). Sorted neutrophils (>99.5% purity by CD11b high Ly6G high expression, Supplementary Fig. 12 ) were suspended at 5 × 10 6 cells ml −1 and then incubated at 37°C in 5% CO 2 atmosphere in the presence or absence of 25 μM R848 or 10 μg ml −1 LPS for 14 h. For in vivo detection of IL-6 production by neutrophils, mice were intraperitoneally injected with BIOgel polyacrylamide beads in the presence of 3 μg g −1 body weight of R848 or its diluent. BIOgel-elicited peritoneal neutrophils were then isolated and either immediately processed for total RNA or protein extraction, or cultured for additional 14 h at high cellular density (10 7 cells ml −1 ). C57BL/6J mice, obtained from Jackson Laboratories (Bar Harbour, ME, USA), were housed under specific pathogen-free conditions at the University of Verona. Experiments were performed with female mice of 8–10 weeks old according to protocols approved by Italian Ministry of Health and in agreement to the current European Community rules on animal protection. Statistical analysis Data are expressed as means±s.e. Statistical evaluation was performed using one-way analysis of variance or two-way analysis of variance followed by Tukey’s or Bonferroni’s post hoc test, respectively. Values of P <0.05 were considered statistically significant. Study approval Human samples were obtained following informed written consent by healthy donors and patients. The study has been cleared by the Ethic Committee of the Azienda Ospedaliera Universitaria Integrata di Verona (Italy). How to cite this article: Zimmermann, M. et al. Chromatin remodelling and autocrine TNFα are required for optimal interleukin-6 expression in activated human neutrophils. Nat. Commun. 6:6061 doi: 10.1038/ncomms7061 (2015).